Active sampling and decision making inDrosophilachemotaxis The ability to respond to chemical stimuli is fundamental to the survival of motile organisms, but the strategies underlying odour tracking remain poorly understood. Here we show that chemotaxis in Drosophila melanogaster larvae is an active sampling process analogous to sniffing in vertebrates. Combining computer-vision algorithms with reconstructed olfactory environments, we establish that larvae orient in odour gradients through a sequential organization of stereotypical behaviours, including runs, stops, lateral head casts and directed turns. Negative gradients, integrated during runs, control the timing of turns. Positive gradients detected through high-amplitude head casts determine the direction of individual turns. By genetically manipulating the peripheral olfactory circuit, we examine how orientation adapts to losses and gains of function in olfactory input. Our findings suggest that larval chemotaxis represents an intermediate navigation strategy between the biased random walks of Escherichia Coli and the stereo-olfaction observed in rats and humans. Animals respond to environmental cues by organizing sequences of movement in space and time. In this process, acquiring sensory information and executing motor responses are intertwined in a continuous feedback loop. Thus, the movement of an animal influences its own sensory experience, inducing motor output, which in turn generates new sensory input. To exploit such feedbacks between sensation and orientation, organisms have evolved sophisticated strategies including chemotaxis, a prominent example of goal-directed behaviour. Bacteria, such as Escherichia Coli , and the nematode, Caenorhabditis elegans , chemotax according to a random walk biased by sensory experience [1] , [2] . Animals with more complex nervous systems show refined scent-tracking strategies. Dogs hunt their prey by moving their nose back and forth across an odour trail [3] and rats use stereo snapshots of the environment through sniffs [4] . In species as different as moths, crustaceans and humans, trail tracking leads to zigzagging trajectories [5] , [6] . Here we study chemotaxis in the fruit fly Drosophila melanogaster . When introduced into an attractive odour gradient, Drosophila larvae migrate towards the direction of higher concentrations. The high precision with which larvae orient up the gradient excludes the involvement of an indirect orientation mechanism such as a biased random walk [7] , [8] . To extract directional information from the environment, larvae may use two strategies: stereo-olfaction and/or spatio-temporal sampling. Earlier, it has been shown that larvae with olfactory function restricted to one side of the head are able to chemotax [8] . In addition, the typical concentration differences measured between the left and right olfactory organs are subject to low copy number fluctuations that places bilateral comparisons close to their physical limits [7] . Accordingly, we hypothesize that larval chemotaxis relies primarily on an active sampling process. During chemotaxis, larvae crawl forward and bend their head sideways. Because the olfactory organs are located at the anterior end of the body, lateral head sweeps (head casts) could lead to the temporal detection of concentration differences between different points in space. To investigate this idea, we developed a new methodology to analyse the time courses of olfactory input that precede the initiation of specific motor outputs. We dissected the sensory-motor algorithm controlling chemotaxis and examined the importance of head casting and stereo-olfaction. Our results indicate that larvae use an active sampling process to detect odour gradients. Reconstructing sensory input from behavioural output Larval chemotaxis was studied in stable odorant environments. As detailed elsewhere [9] , we devised odour gradients with controllable properties in small arenas. We then reconstructed the geometry of these gradients by using a fast-Fourier infrared spectroscopy technique [8] . In our assays, larvae were not tethered nor exposed to discrete odour puffs or turbulent plumes, but instead they freely explored static gradients ( Fig. 1a ). Combined with a quantitative knowledge of the stimulus conditions, we tracked behaviour at a resolution beyond the commonly used centroid (geometric centre) description. We developed a computer-vision tracking system, which captures the posture of freely moving larvae in real time and at a high-spatial resolution ( Supplementary Movie 1 ). Following ref. 10 , we devised an algorithm for the automated extraction of the larva's centreline and the identification of four loci of interest: the larva's head, tail, midpoint and centroid ( Fig. 1b ). In this process, we converted larval images into a set of kinematic variables that capture relevant body postural dynamics. 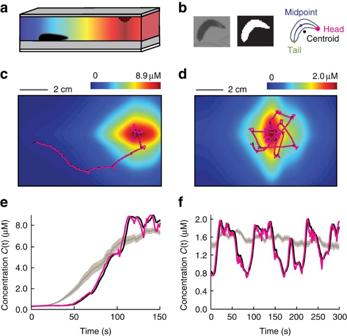Figure 1: High-resolution measurements of sensory input and motor output. (a) Representation of the behavioural assay forDrosophilalarval chemotaxis. (b) Schematic of the automated computer-vision tracking algorithm. (c) Fourier transform infrared spectroscopy reconstruction of the odour gradient overlaid with a representative trajectory of the head (magenta) and the centroid (black) while approaching a 125 mM source of ethyl butyrate. (d) Same as for (c) when orbiting near a 30 mM odour source. (e) Concentration time course measured at the head and centroid positions corresponding to the representative trajectory in (c). Population-averaged head concentration represented in the background as a grey curve (mean±s.e.m.,N=43 flies). (f) Same as for (e) in the near-source conditions of (d) (N=42). Figure 1: High-resolution measurements of sensory input and motor output. ( a ) Representation of the behavioural assay for Drosophila larval chemotaxis. ( b ) Schematic of the automated computer-vision tracking algorithm. ( c ) Fourier transform infrared spectroscopy reconstruction of the odour gradient overlaid with a representative trajectory of the head (magenta) and the centroid (black) while approaching a 125 mM source of ethyl butyrate. ( d ) Same as for ( c ) when orbiting near a 30 mM odour source. ( e ) Concentration time course measured at the head and centroid positions corresponding to the representative trajectory in ( c ). Population-averaged head concentration represented in the background as a grey curve (mean±s.e.m., N =43 flies). ( f ) Same as for ( e ) in the near-source conditions of ( d ) ( N =42). Full size image We studied the ability of freely moving Drosophila larvae to locate and to remain in the vicinity of an attractive odour source. A single source of ethyl butyrate—a fruity ester abundant in citrus and pineapple—was suspended from the top of the arena at a position out of the larva's reach. Individual larvae placed at the opposite end of the plate successfully ascended the gradient ( Supplementary Movie 2 ). The representative trajectory shown in Figure 1c illustrates that this behaviour consists of two steps: an approach phase and a near-source phase. The near-source behaviour involves frequent turns as larvae reach, overshoot and return to the odour source. Animal starting under the source created 'ball-of-wool-like' trajectories ( Fig. 1d ). We reconstructed the time course of the concentration experienced by the animal's head (magenta) and centroid (black) along their trajectories ( Fig. 1e,f ). Fluctuations in concentration are typically larger at the head than at the centroid. Following the hypothesis that orientation is guided by spatio-temporal sampling, we expected behavioural responses to be controlled by temporal changes in the perceived stimulus intensity at the tip of the head. As with other sensory modalities, we assumed that changes in perception (Δ ψ ) are related to changes in physical stimulus (Δ C ) by the Weber–Fechner law [11] . Accordingly, perceived changes in odour concentration are assumed to be proportional to the logarithm of stimulus increases, Δ ψ ~ln(Δ C ). Therefore, our proxy for the signal that a larva extracts from the environment is 1/ C ·d C /dt. This quantity represents an amplitude-normalized measure of the temporal changes in concentration. To correlate changes in sensory input with behavioural states, we defined a set of relevant kinematic variables describing the movement, posture and orientation of a larva in the odour gradient: the locomotion speed v centroid , the head speed v head , the direction of locomotion or body angle α , the instantaneous reorienation speed d α /d t , the head angle θ between the body and neck axis, and the alignment of the animal with the local odour gradient quantified by the bearing angle β ( Fig. 2 and Methods). 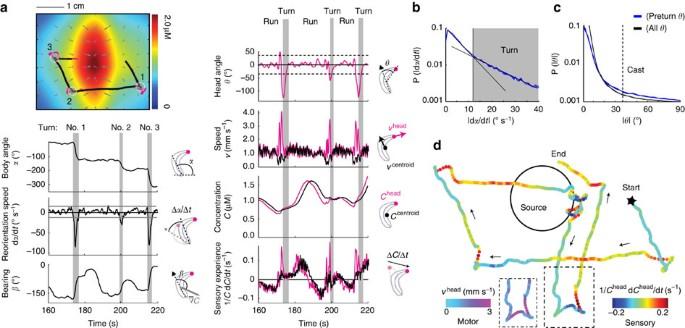Figure 2: Kinematic variables and behavioural states. (a) Trajectory segment in an odour gradient field and temporal evolution of its associated sensory-motor variables: body angle orientation (α), reorientation speed (dα/dt), bearing (β) of the animal with respect to the local odour gradient, head angle (θ), head and centroid speed (v), odour concentration (C) at the head and centroid, and temporal concentration changes (1/C·dC/dt) capturing sensory experience. Occurrence of turns (grey circles numbered from 1 to 3 in the trajectory segment) is indicated by vertical grey bars. (b) Definition of turns. The crossover in the reorientation speed distribution of the wild-type dataset (blue curve) provides a natural threshold to define turns (grey region) as |dα/dt|>ω*(ω*=12° s−1, see grey line in (a) for the reorientation speed). Dashed lines indicate estimated counting errors of the distributions based on a bootstrapping procedure. (c) Definition of head casts. The distribution of head angle across the wild-type dataset (black curve) is compared with the distribution obtained from the 4 s preceding a turn (blue curve). Large fluctuations in head angle are more frequent immediately before a turn, which allows to define discrete head casts as peaks in head angle for which |θ|>θ*(θ*=37°, see also dotted line in (a) for head angle). (d) Illustrative trajectory of the reconstructed concentration changes experienced by the head of a freely moving larva. The inset depicts head speed. As illustrated in Figure 2a , trajectories are approximately piecewise and can be parsed into segments of straight locomotion (runs) interspersed with abrupt orientation changes (turns). Fast reorientation events are defined as turns ( Fig. 2b ). Likewise, large bends in the animal's posture are defined as head casts ( Fig. 2c ). The set of continuous variables and discrete states shown in Figure 2a–c allows us to comprehensively quantify stimulus input and behavioural output. Figure 2d illustrates the relationship between sensory experience, head motion and orientation behaviour during navigation near the odour source. Figure 2: Kinematic variables and behavioural states. ( a ) Trajectory segment in an odour gradient field and temporal evolution of its associated sensory-motor variables: body angle orientation ( α ), reorientation speed (d α /d t ), bearing ( β ) of the animal with respect to the local odour gradient, head angle ( θ ), head and centroid speed ( v ), odour concentration ( C ) at the head and centroid, and temporal concentration changes (1/ C ·d C /dt) capturing sensory experience. Occurrence of turns (grey circles numbered from 1 to 3 in the trajectory segment) is indicated by vertical grey bars. ( b ) Definition of turns. The crossover in the reorientation speed distribution of the wild-type dataset (blue curve) provides a natural threshold to define turns (grey region) as |d α /d t |> ω *( ω *=12° s −1 , see grey line in ( a ) for the reorientation speed). Dashed lines indicate estimated counting errors of the distributions based on a bootstrapping procedure. ( c ) Definition of head casts. The distribution of head angle across the wild-type dataset (black curve) is compared with the distribution obtained from the 4 s preceding a turn (blue curve). Large fluctuations in head angle are more frequent immediately before a turn, which allows to define discrete head casts as peaks in head angle for which |θ|>θ*(θ*=37°, see also dotted line in ( a ) for head angle). ( d ) Illustrative trajectory of the reconstructed concentration changes experienced by the head of a freely moving larva. The inset depicts head speed. Full size image Larvae are able to orient in the direction of the gradient Localizing and staying near the odour source implies a controlled alternation between runs and turns. But, when is a run terminated and how is the direction of the following turn determined? To address these two questions, we analysed the bearing angle distribution of wild-type larvae before each turn initiation ( Fig. 3a ). We found that 81.6% (±1.1% s.e.m.) of turns were triggered at down-gradient orientations (| β |>90 degrees, Fig. 3b ). This demonstrates that larvae are capable of detecting decreases in concentration during forward locomotion. By comparing the change in bearing before and after each turn, we found that 73.9% (±1.3% s.e.m.) of turns reorient the larva towards higher odour concentrations. Furthermore, grouping bearing angles before a turn according to the direction of reorientation ( Fig. 3c ) revealed that larvae can resolve whether the gradient is pointing to their left or to their right side. Therefore, larvae control both the timing and direction of their turns. Whereas individual turns tend to undershoot the direction of the gradient ( Fig. 3d ), consecutive turns permit larvae to reach the odour source and to stay in its vicinity. Asymmetries in the local odour distribution are largest for bearing angles close to 90° and smallest at 180° where lateral head casts lead to poorly contrasted concentration differences. We found that turns towards the direction of lower concentrations correspond to initial orientations where the larva stood with the source in their back ( Fig. 3e ). Reorientation performances are optimal when larvae are aligned perpendicularly to the gradient ( Fig. 3f ). 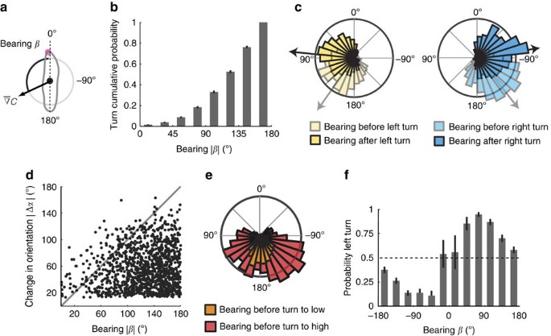Figure 3: Temporal and directional control of turning events. (a) Schematic representation of larval bearing with respect to the local odour gradient. (b) Cumulative probability of turns as a function of the absolute bearing angle. Turns are more likely to be triggered when larvae navigate down-gradient (|β|>90°). Error bars indicate s.e.m. (c) Distributions of bearing angles before (translucid) and after (opaque) turns, constrained to left (yellow) and right (blue) reorientations. (d) Absolute change in body orientation angle during turning events (|Δα|) as a function of the absolute bearing angle before turn initiation (|β|). Whereas larvae seem unable to precisely estimate the exact value of the bearing angle, the majority of turns do not overshoot the direction of the local gradient (diagonal). (e) Bearing distributions for turns towards high and low. Turns towards low are initiated at down-gradient orientations where spatial asymmetries in the odour gradient are more difficult to resolve via lateral head casts. (f) Probability to turn towards the left side as a function of the bearing before turn initiation. Vertical bars represent s.e.m. The accuracy of a turn is optimal for bearing close to 90°, where the odour gradient is perpendicular to the larva. For bearing angles close to 180 degrees, the turning direction tends to be random. For all panels,N=1,243 turns. Figure 3: Temporal and directional control of turning events. ( a ) Schematic representation of larval bearing with respect to the local odour gradient. ( b ) Cumulative probability of turns as a function of the absolute bearing angle. Turns are more likely to be triggered when larvae navigate down-gradient (| β |>90°). Error bars indicate s.e.m. ( c ) Distributions of bearing angles before (translucid) and after (opaque) turns, constrained to left (yellow) and right (blue) reorientations. ( d ) Absolute change in body orientation angle during turning events (|Δ α |) as a function of the absolute bearing angle before turn initiation (| β |). Whereas larvae seem unable to precisely estimate the exact value of the bearing angle, the majority of turns do not overshoot the direction of the local gradient (diagonal). ( e ) Bearing distributions for turns towards high and low. Turns towards low are initiated at down-gradient orientations where spatial asymmetries in the odour gradient are more difficult to resolve via lateral head casts. ( f ) Probability to turn towards the left side as a function of the bearing before turn initiation. Vertical bars represent s.e.m. The accuracy of a turn is optimal for bearing close to 90°, where the odour gradient is perpendicular to the larva. For bearing angles close to 180 degrees, the turning direction tends to be random. For all panels, N =1,243 turns. Full size image Turns are triggered after stereotypical olfactory signals To establish the orientation mechanisms maintaining a larva aligned with the odour gradient, we analysed the average sensory-motor history preceding a turn. The turn-triggered average of the animal's speed ( Fig. 4a ) shows that turning is preceded by a transient reduction of forward locomotion, which lasts 1–3 s. During that episode, a large increase in the head speed is observed. As locomotion is interrupted before turning, peaks in head speed are not part of a wave of peristaltic contraction: they correspond to head casts that generate contrasted changes in relative odour concentration. 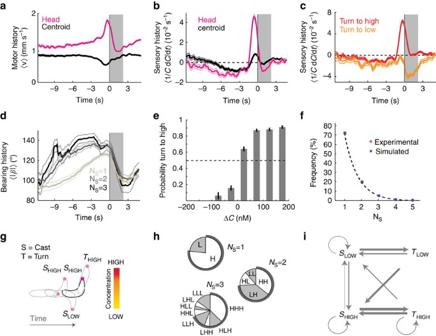Figure 4: Stereotypical sensory-motor history associated with casts and turns. (a) Turn-triggered averages of head and centroid speed (mean±s.e.m.). Grey bar shading in the turn-triggered plots indicate turning. (b) Average perceived changes in odour concentration aligned with turn initiation. Concentration decreases (negative values) precede the transition from run to turn. Turn initiation follows abrupt positive temporal changes in concentration measured at the head position. High-amplitude positive peaks are caused by active sampling during head casting. (c) Turn-triggered average of perceived stimulus changes clustered by turns towards high and low. Turns directed towards high are preceded by large stimulus increases. Turns directed towards low are preceded by low-contrast stimulus experiences. (d) Average time course of the bearing angle aligned with turn onset. The larger the bearing angle history before the turn, the larger the number of head casts (NS) before the implementation of a turn. (e) Probability to turn towards high as a function of the concentration change (ΔC) experienced during the last head cast before turning. Error bars indicate s.e.m. (f) Histogram of the number of head casts observed before turn execution. The distribution follows a negative exponential function (dashed line). (g) Diagram of the cast-and-turn motor dynamics coupled with a high-or-low sensory experience description. (h) Pie charts of head casting pattern sequences before turning calculated on experimental data: bouts of head cast towards high (H) and towards low (L). Head cast towards low concentrations is often followed by another head cast towards high. Patterns ending on high dominate. (i) Ethogram classification of odour-search behaviour into four elementary 'action–perception' states: turns (T) and head casts (S) towards low (L) and high (H). Illustration of the 4 behavioural states of the model. Transition probabilities between states calculated on the basis of a first-order Markov chain trained on the experimental data. Arrow thicknesses are proportional to the transition probabilities. Numerically simulated sequences of state transitions show an excellent fit with the experimentally measured exponential distribution of the number of head casts. For all panels,N=1,243 turns. As shown in Figure 4b , the turn-triggered average of the perceived change in odour concentration steadily declines from positive values (concentration increasing) to negative values (concentration decreasing), crossing zero about 8 s before the turn starts. This stereotypical decrease in concentration appears to be the signal that terminates a run, triggers head casting and initiates a turn. Figure 4: Stereotypical sensory-motor history associated with casts and turns. ( a ) Turn-triggered averages of head and centroid speed (mean±s.e.m.). Grey bar shading in the turn-triggered plots indicate turning. ( b ) Average perceived changes in odour concentration aligned with turn initiation. Concentration decreases (negative values) precede the transition from run to turn. Turn initiation follows abrupt positive temporal changes in concentration measured at the head position. High-amplitude positive peaks are caused by active sampling during head casting. ( c ) Turn-triggered average of perceived stimulus changes clustered by turns towards high and low. Turns directed towards high are preceded by large stimulus increases. Turns directed towards low are preceded by low-contrast stimulus experiences. ( d ) Average time course of the bearing angle aligned with turn onset. The larger the bearing angle history before the turn, the larger the number of head casts (N S ) before the implementation of a turn. ( e ) Probability to turn towards high as a function of the concentration change (Δ C ) experienced during the last head cast before turning. Error bars indicate s.e.m. ( f ) Histogram of the number of head casts observed before turn execution. The distribution follows a negative exponential function (dashed line). ( g ) Diagram of the cast-and-turn motor dynamics coupled with a high-or-low sensory experience description. ( h ) Pie charts of head casting pattern sequences before turning calculated on experimental data: bouts of head cast towards high (H) and towards low (L). Head cast towards low concentrations is often followed by another head cast towards high. Patterns ending on high dominate. ( i ) Ethogram classification of odour-search behaviour into four elementary 'action–perception' states: turns ( T ) and head casts ( S ) towards low (L) and high (H). Illustration of the 4 behavioural states of the model. Transition probabilities between states calculated on the basis of a first-order Markov chain trained on the experimental data. Arrow thicknesses are proportional to the transition probabilities. Numerically simulated sequences of state transitions show an excellent fit with the experimentally measured exponential distribution of the number of head casts. For all panels, N =1,243 turns. Full size image While vigorously sweeping their head on one side, larvae experience typical increases in concentration of 100 nM ( Supplementary Fig. S1 ). This process permits larvae to extract directional information from their surroundings to direct a turn. The peak in sensory experience, also observed in the turn-triggered average of the non-normalized time derivative of the concentration d C /d t ( Supplementary Fig. S2 ), is not a simple consequence of the turning maneuver. Grouping cases where turns orient the larva towards higher concentrations (up-gradient) or lower concentrations (down-gradient) reveals that a large peak in sensory experience is predictive of reorientations towards higher concentrations ( Fig. 4c ). Turns towards low tend to follow head casts leading to non-significant concentration increases before turn initiation. Furthermore, in conditions of poorly contrasted olfactory experience, the number of head casts increases before the initiation of a turn ( Fig. 4d ). Whenever the last head cast is associated with a concentration increase larger than 50 nM, the likelihood of turning to high exceeds 80% ( Fig. 4e ). Turns are directed by active sampling relying on head casts The distribution of the natural number of head casts preceding a turn ( N S ) follows a negative exponential function ( Fig. 4f ). Turning events associated with more than three head casts are rare. Adopting a binary description, we classified head casts into two categories: sweeps towards higher (H) or lower (L) concentrations ( Fig. 4g ). Because the body follows the head during forward peristalsis, the last head cast determines the direction of the turn. We found that larvae are capable of identifying the direction of increasing concentrations in more than 70% of cases within the first two head casts ( Fig. 4h ). A first head cast towards low is likely to be followed by a second head cast towards high (pattern 'LH'). Conversely, a head–cast-to-high rarely triggers a second head cast towards the opposite direction. We built a first-order Markov model to investigate the relevance of high-order memory effects in the transition dynamics between consecutive head casts and turns. Considering four action–perception states (head cast to low ( S LOW ) and to high ( S HIGH ), turn to low ( T LOW ) and to high ( T HIGH )), the matrix of transition probabilities between states was obtained by training the model with the experimental transition sequences of wild-type larvae. The connected graph in Figure 4i is a probabilistic representation of the dynamics inherent to the sampling and turning processes controlling chemotaxis. The thickness of each edge is proportional to the probability of that transition. Next, we simulated sequences of state transition with a Monte Carlo algorithm based on the experimental probability transition matrix. The fitness of the model was assessed by comparing the experimental and simulated frequency distributions of the number of head cast preceding a turn ( Fig. 4f ) together with the frequency of individual head cast patterns ( Supplementary Fig. S3 ). The excellent agreement between the model and the experimental data suggests that the decision-making process does not necessarily involve high-order memory effects. Only the sensory-motor experience associated with the most recent turn appears to influence the next head-casting episode. On average, nearly 70% of turns are preceded by a first head cast towards high. Together, our findings indicate that the direction of the first head cast is not selected at random. Larvae have a mechanism to bias their sampling towards the direction of the gradient. Manipulation of olfactory input To elucidate the neural computation controlling chemotaxis, we genetically modified the peripheral olfactory circuit to produce losses and gains of olfactory input ( Fig. 5a ). The larval olfactory system is composed of two bilaterally symmetrical organs called dorsal organs. Each organ hosts 21 olfactory receptor neurons (ORNs) [12] . Every ORN expresses a single type of 'private' olfactory receptor together with the 'public' co-receptor Orco (previously named Or83b ) [13] , [14] , [15] . Olfactory function is abolished in mutants lacking Orco expression [16] . Individual ORNs are tuned to different classes of odours and different concentration ranges. Among all olfactory receptors expressed at the larval stage, the three receptors with the highest affinity to ethyl butyrate are Or35a , Or42a and Or42b (ref. 13 ). We examined how manipulating the input provided by the Or42a receptor impacts on olfactory navigation, active sampling and reorientation performances. 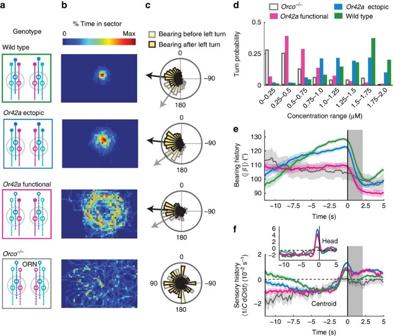Figure 5: Navigational algorithm adaptation to genetic manipulations of peripheral olfactory inputs. (a) Schematic of wild type and larvae with re-engineered peripheral olfactory circuits tested in the near-source paradigm (30 mM odour source): wild type (N=42 flies),Or42aectopically expressed in the 21 intact ORNs (all neuron pairs active,N=38),Or42asingle-functional ORN (one pair of neuron active,N=37), andOrconull (anosmic flies,N=55). (b) Time occupancy spatial maps (4 mm2sectors) for each tested genotype. (c) Distribution of bearing angles before and after turns towards left. Circular means of bearings before (grey) and after (black) turns are represented as arrows. The amplitude of reorientation is modulated across genotypes. (d) Turning probability as a function of odour concentration.Or42a-ectopic larvae (N=951 turns) implement turns over a wider range of concentrations, whereasOr42a-functional (N=533) turn at much lower concentrations than wild type (N=1,243). (e) Turn-triggered averages of bearing angle (mean±s.e.m.). Grey bars indicate turns. (f) Comparison of turn-triggered sensory experience across genotypes. WhereasOr42a-ectopic larvae display the same trend as wild type with a reduced slope,Or42a-functional larvae tend to maintain a constant negative value. Figure 5: Navigational algorithm adaptation to genetic manipulations of peripheral olfactory inputs. ( a ) Schematic of wild type and larvae with re-engineered peripheral olfactory circuits tested in the near-source paradigm (30 mM odour source): wild type ( N =42 flies), Or42a ectopically expressed in the 21 intact ORNs (all neuron pairs active, N =38), Or42a single-functional ORN (one pair of neuron active, N =37), and Orco null (anosmic flies, N =55). ( b ) Time occupancy spatial maps (4 mm 2 sectors) for each tested genotype. ( c ) Distribution of bearing angles before and after turns towards left. Circular means of bearings before (grey) and after (black) turns are represented as arrows. The amplitude of reorientation is modulated across genotypes. ( d ) Turning probability as a function of odour concentration. Or42a -ectopic larvae ( N =951 turns) implement turns over a wider range of concentrations, whereas Or42a- functional ( N =533) turn at much lower concentrations than wild type ( N =1,243). ( e ) Turn-triggered averages of bearing angle (mean±s.e.m.). Grey bars indicate turns. ( f ) Comparison of turn-triggered sensory experience across genotypes. Whereas Or42a -ectopic larvae display the same trend as wild type with a reduced slope, Or42a -functional larvae tend to maintain a constant negative value. Full size image First, we ectopically expressed the Or42a odorant receptor in all ORNs. We found that Or42a -ectopic larvae disperse under the source more broadly than wild type. Although they do not accumulate at a fixed distance from the source ( Fig. 5b ), their average bearing before turning is more narrowly distributed around 90° than in wild type ( Fig. 5c ). On average, turns reorient larvae towards the gradient. The distribution of turning frequency shows that turns are triggered for a broader range of concentration in Or42a -ectopic larvae ( Fig. 5d ). When compared with wild type, Or42a -ectopic larvae experience a negative stimulus for a longer period of time before a turn is triggered ( Fig. 5e,f ). The delay in turn triggering suggests that ectopic expression of Or42a in all ORNs modifies the sensory control of transitions from run to turn. Second, we analysed the orientation behaviour of larvae with olfactory input restricted only to the Or42a -expressing ORN [8] . In contrast with wild type, Or42a -functional larvae followed a concentration path distant from the source ( Fig. 5b ; Supplementary Movie 3 ). Here we demonstrate that, to orbit around the source, Or42a -functional larvae implement small-amplitude turns, which maintain their bearing close to 90° ( Fig. 5c ). This result indicates that Or42a -functional larvae are capable of modulating the amplitude of their turns. Turns are triggered at concentrations three times lower than wild type ( Fig. 5d ). However, the targeted concentration does not coincide with the region where the amplitude of the gradient is maximal: the mean gradient slope experienced by the Or42a -functional trajectories is 0.043 μM mm −1 (±0.021 s.e.m. ), whereas the maximum value of the gradient in the arena is 0.13 μM mm −1 . When analysing the turn-triggered average histories of bearing, we found that, in contrast to wild type, turns are preceded by episodes where the bearing remains constant ( Fig. 5e ). As shown in Figure 5f , Or42a -functional larvae undergo a constant change in perceived stimulus whereas wild type larvae experience a monotonic decrease. To test whether Or42a -functional actively avoid areas of high odour concentrations, we studied the orientation behaviour of Or42a -functional approaching a source of ethyl butyrate at low (7.8 mM) and high (125 mM) concentrations. For the low-concentration source ( Fig. 6a ), Or42a -functional larvae show attraction throughout the gradient's range, and accumulate near the source. At high concentrations ( Fig. 6b ), Or42a -functional navigate up-gradient, before they bifurcate to avoid regions of high-odour intensities. In contrast, wild-type larvae display invariant attraction to low and high concentrations. To establish the existence of a switch between attractive and repulsive responses in Or42a -functional, we quantified the probability of turning towards the gradient for different concentration ranges. We found that wild type turn towards the direction of higher concentrations everywhere, except at positions where the absolute concentration was very low ( Fig. 6c ). On the other hand, Or42a -functional larvae turn towards the gradient for concentrations lower than 0.5 μM, but away from the gradient for higher concentrations ( Fig. 6c ). This observation supports a model where the activity conveyed by the Or42a -expressing ORN saturates at high odour concentration [17] . At concentrations within the dynamic range of the Or42a ORN, the stimulus elicits an attractive response. At high concentrations exceeding the dynamic range of the Or42a ORN, the stimulus elicits active avoidance. 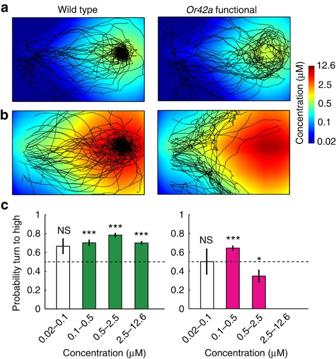Figure 6: Concentration-dependent switch between attraction and avoidance inOr42a-functional larvae. (a) Wild type (N=43 flies) andOr42a-functional (N=42) trajectories superimposed on the concentration landscape reconstructed for the approach paradigm at a low-concentration source of ethyl butye (7.8 mM). Heat map displayed in logarithmic scale. (b) Same as for (a) with wild type (N=43) andOr42a-functional (N=42) tested in a low-concentration source (125 mM) gradient. (c) Probability of turning to high as a function of the concentration range. For absolute odour concentrations lower than 100 nM, turns lead to randomized reorientation. Wild type (N=1,172 turns) show attraction at all other concentration ranges, whereasOr42a-functional (N=455) switch from attraction to avoidance at concentrations close to 500 nM. Error bars indicate s.e.m. Differences of turning probabilities with chance were tested by a one-tailed one-samplet-test (*P<0.05; ***P<0.001; NS, not significantP>0.05). Figure 6: Concentration-dependent switch between attraction and avoidance in Or42a -functional larvae. ( a ) Wild type ( N =43 flies) and Or42a -functional ( N =42) trajectories superimposed on the concentration landscape reconstructed for the approach paradigm at a low-concentration source of ethyl butye (7.8 mM). Heat map displayed in logarithmic scale. ( b ) Same as for ( a ) with wild type ( N =43) and Or42a -functional ( N =42) tested in a low-concentration source (125 mM) gradient. ( c ) Probability of turning to high as a function of the concentration range. For absolute odour concentrations lower than 100 nM, turns lead to randomized reorientation. Wild type ( N =1,172 turns) show attraction at all other concentration ranges, whereas Or42a -functional ( N =455) switch from attraction to avoidance at concentrations close to 500 nM. Error bars indicate s.e.m. Differences of turning probabilities with chance were tested by a one-tailed one-sample t -test (* P <0.05; *** P <0.001; NS, not significant P >0.05). Full size image Finally, we genetically manipulated the signal-to-noise ratio in the detection of small concentration changes by engineering larvae with olfactory function restricted to a single unilateral Or42a -expressing ORN. As shown earlier, unilateral function does not produce a significant decrease in sensory threshold to ethyl butyrate [8] . Both larvae with bilateral and unilateral function in the Or42a ORN tend to orbit around the source. Here we observe that larvae with unilateral function navigate more poorly and display tortuous paths ( Fig. 7a ). When compared with bilateral, unilateral function leads to subtle differences in the turn-triggered average time courses of the bearing and the perceived stimulus change. The mean bearing angle before turning is higher for unilateral than bilateral larvae, suggesting a reduction in the ability of unilateral to maintain a fixed orbit ( Fig. 7b ). Likewise, the perceived stimulus change switches earlier from a constant negative value to positive values, indicating higher sampling activity in unilateral larvae before turning ( Fig. 7b ). We observed no side bias in head casting direction between unilateral left and right larvae ( Fig. 7c ). Finally, we quantified the ability of unilateral and bilateral larvae to reorient towards the gradient for concentrations sufficiently low to elicit pure attraction (C<500 nM, Fig. 6c ). We found no difference between the probabilities of turning high in unilateral left and right larvae (one-tailed two-sample t -test, P =0.49, number of turns N =70 and N =95 for unilateral left and right, respectively). Whereas larvae with unilateral function fail to robustly orient towards the gradient, bilateral olfactory function permits them to direct their turns towards higher concentrations ( Fig. 7d ). We hypothesize that unilateral function is likely to be associated with larger perceptual uncertainties owing to noisier assessments of concentration differences during head casting. On the whole, unilateral function in Or42a ORN does not abolish, but reduces the active sampling accuracy. Bilateral function provides an advantage in the integration of concentration differences during runs and head casts. 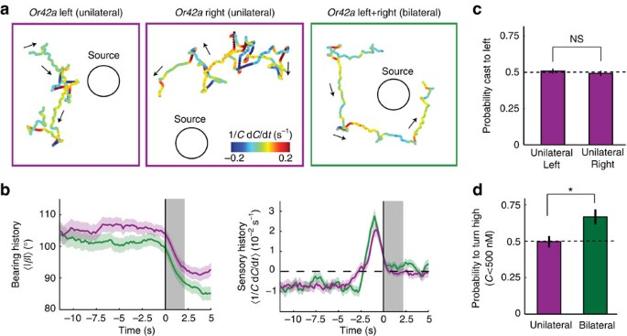Figure 7: Impairment of bilateral olfactory function reduces navigational accuracy. Or42a-functional larvae with olfactory function restricted to the left side (N=47 flies), the right side (N=47), and both sides (N=56). (a) Representative trajectories of the reconstructed concentration time course measured at the head. (b) Turn-triggered average history of the bearing angle inOr42a-functional larvae with unilateral and bilateral functions (mean±s.e.m.). Grey bar shading indicates turning event. Unilateral tend to initiate turns for bearing larger than bilateral, suggesting a less reliable assessment of stimulus time course. Turn-triggered average history of perceived stimulus change at the head. The constant negative trend in unilateral larvae is interrupted earlier than in bilateral larvae, leading to higher active sampling activity before turn execution. (c) Unilateral left (N=848 casts) and right (N=714) larvae do not show biases in the probability of head casting towards the left side (one-tailed one-samplet-test against chance,P=0.68 andP=0.63 for left and right, respectively). In addition, the performances of unilateral left and right are not significantly different (one-tailed two-samplet-test,P=0.53). Error bars indicate s.e.m. (d) The probability of implementing a turn towards high at low concentrations is above chance in bilateral larvae (one-tailed one-samplet-test,P=0.002), whereas it is not significantly different from chance for unilateral larvae (one-tailed one-samplet-test,P=0.94). The performance of bilateral larvae are significantly higher than those of unilateral (one-tailed two-samplet-test,P=0.011, *P<0.05). Number of turns at positions where C<500 nM:N=165 for pooled unilateral andN=84 for bilateral. Figure 7: Impairment of bilateral olfactory function reduces navigational accuracy. Or42a -functional larvae with olfactory function restricted to the left side ( N =47 flies), the right side ( N =47), and both sides ( N =56). ( a ) Representative trajectories of the reconstructed concentration time course measured at the head. ( b ) Turn-triggered average history of the bearing angle in Or42a -functional larvae with unilateral and bilateral functions (mean±s.e.m.). Grey bar shading indicates turning event. Unilateral tend to initiate turns for bearing larger than bilateral, suggesting a less reliable assessment of stimulus time course. Turn-triggered average history of perceived stimulus change at the head. The constant negative trend in unilateral larvae is interrupted earlier than in bilateral larvae, leading to higher active sampling activity before turn execution. ( c ) Unilateral left ( N =848 casts) and right ( N =714) larvae do not show biases in the probability of head casting towards the left side (one-tailed one-sample t -test against chance, P =0.68 and P =0.63 for left and right, respectively). In addition, the performances of unilateral left and right are not significantly different (one-tailed two-sample t -test, P =0.53). Error bars indicate s.e.m. ( d ) The probability of implementing a turn towards high at low concentrations is above chance in bilateral larvae (one-tailed one-sample t -test, P =0.002), whereas it is not significantly different from chance for unilateral larvae (one-tailed one-sample t -test, P =0.94). The performance of bilateral larvae are significantly higher than those of unilateral (one-tailed two-sample t -test, P =0.011, * P <0.05). Number of turns at positions where C<500 nM: N =165 for pooled unilateral and N =84 for bilateral. Full size image Over the past century, many studies have documented a variety of phenomenological rules directing behaviour in response to light, sounds and chemicals [18] . Goal-oriented behaviours have been the subject of increasing attention in Drosophila . Recent technological advances have permitted fly neurobiologists to investigate how visual cues are integrated with mechano-sensory feedbacks in tethered and freely flying flies [19] , [20] . Orientation in response to such inputs has also been examined in walking flies driven by a stripe or engaged in gap crossing [21] , [22] . Due to difficulties inherent in the measurement of odour diffusion in gaseous phase, the analysis of odour-tracking behaviours has lagged behind the functional characterization of olfactory systems [23] . Our work bridges this long-standing gap between the functional characterization of the fly olfactory system and naturalistic orientation behaviour. We have developed a computer-vision algorithm to monitor the behaviour of freely moving larvae. By correlating sensory input and behavioural output at a high spatio-temporal resolution, we uncovered the chief mechanisms enabling Drosophila larvae to navigate in odour gradients. 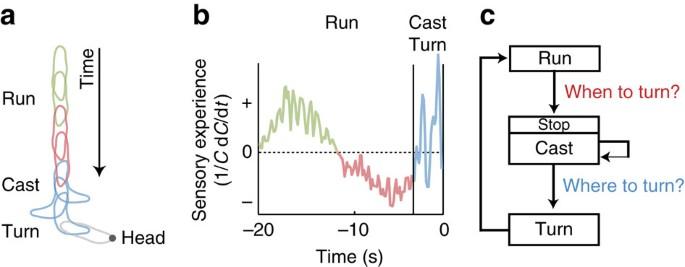Figure 8: Sensory-motor model for larval chemotaxis. (a) Schematic of a trajectory segment consisting of a run followed by a turn. The sequence of body postures corresponds to forward locomotion oriented up-gradient (green) and down-gradient (red) followed by a series of head casts (blue) and a turn (gray). (b) Sensory experience associated with the trajectory segment depicted in (a). During up-gradient motion (green), the sensory experience detected at the larva's head region is positive. On motion down-gradient (red), the sensory experience is negative for several seconds, which triggers a transition from running to head casting (blue). Head casts are associated with short and contrasted changes in odour concentration. (c) Diagram of the basic computation and rules controlling larval navigation in odour gradients. Chemotaxis consists of two main types of decision: when and where to turn. Temporal control of transitions from run to turn implies low-pass filtering, differentiation and time integration of sensory input measured during forward locomotion. The directional control of individual turns is mediated by an active sampling mechanism based on head casting. As described in Figure 8 , larval chemotaxis entails two main types of decision: controlling the timing of turning event (when to turn), and directing individual turns with respect to the local odour gradient (where to turn). We found that both types of decisions involve active sampling where information about the olfactory environment is collected during stereotypical patterns of behaviour. Like C. elegans , Drosophila larvae appear to low-pass filter, differentiate, integrate and compare olfactory inputs [2] . During runs, the integration of monotonic decreases in concentration triggers a turn (long timescale, greater than 5 s). Before turning, rapid head casts resolve spatial asymmetries in the surrounding odour gradients (short timescale, smaller than 1 s), which permit larvae to direct their turns towards the direction of higher concentrations. Figure 8: Sensory-motor model for larval chemotaxis. ( a ) Schematic of a trajectory segment consisting of a run followed by a turn. The sequence of body postures corresponds to forward locomotion oriented up-gradient (green) and down-gradient (red) followed by a series of head casts (blue) and a turn (gray). ( b ) Sensory experience associated with the trajectory segment depicted in ( a ). During up-gradient motion (green), the sensory experience detected at the larva's head region is positive. On motion down-gradient (red), the sensory experience is negative for several seconds, which triggers a transition from running to head casting (blue). Head casts are associated with short and contrasted changes in odour concentration. ( c ) Diagram of the basic computation and rules controlling larval navigation in odour gradients. Chemotaxis consists of two main types of decision: when and where to turn. Temporal control of transitions from run to turn implies low-pass filtering, differentiation and time integration of sensory input measured during forward locomotion. The directional control of individual turns is mediated by an active sampling mechanism based on head casting. Full size image Many arthropods exploit the detection of small concentration differences between bilateral olfactory sensors (stereo-olfaction) to locate the source of an attractive smell [24] , [25] , [26] , [27] . Walking adult flies turn in response to concentration differences measured across their antennae [28] . In the absence of inter-antennal gradient, the orientation strategy of honeybees switches from instantaneous comparisons of bilateral olfactory inputs to temporal sampling mediated by zigzagging runs [29] . In line with previous work [8] , we found that stereo-olfaction is not required for larvae to control the onset of turning, but that bilateral olfactory input enhances turning performances ( Fig. 7d ). This result corroborates the idea that detecting minute concentration changes during head casting is facilitated by the use of two independent sensors [7] . We also discovered that the frequency of head casting increases when an individual fails to gather reliable evidence about the direction of the gradient ( Fig. 4d ). Finally, comparing the reorientation strategies of wild type and Or42a -functional larvae led us to conclude that larvae modulate the amplitude of their turns in a task-dependent manner. In the extreme case where the stimulus intensity exceeds the coding capacity of the peripheral olfactory system, innate attraction to the odour is converted into active avoidance ( Fig. 6 and ref. 17 ). Our work illustrates how a complex behaviour emerges from a series of elementary actions: runs, stops, head casts and turns. Several lines of evidence suggest that a similar behavioural hierarchy contributes to the orientation responses elicited by other sensory modalities [30] , [31] , [32] . We showed that the strategy used by Drosophila larvae is not reducible to the improved biased random walk of E. coli and the error-compensation strategy of C. elegans [2] , [7] . Instead, head casting in larvae constitutes an active sampling mechanism analogous to 'sniffing' in higher-order animals [33] . A 'sniff' can be defined as a brief increase in air or water flow across the olfactory organ. Whereas vertebrates draw repetitive air samples through their nasal cavities [34] , [35] , insects and crustaceans flick their antennae [36] , [37] , [38] . During a sniff—whether it corresponds to inhalation or antennal flick—the volume of fluid surrounding the olfactory organ is replaced, which provides the animal with a new sample of its olfactory environment. Sniffing also increases the interception rate of odorants molecules by the olfactory neurons—a phenomenon achieved by wing flapping in moths and adult flies [36] , [39] , [40] . Our results indicate that larvae use head casting to punctuate the processing of their olfactory environment. During a head cast, larvae detect variations in odour concentration with a contrast enhanced by the rapid translation of the sensors located at the tip of the head. Even though the potential involvement of peripheral adaption will need to be clarified further, we speculate that head casting relies on short-term memorization that enables a central comparison of stimulus changes measured during successive head casts. A similar mechanism is thought to underlie goal-directed behaviour in adult flies [21] . In analogy to rats and humans, which associate exploratory head movements with stereo snapshots of the environment [4] , [5] , [34] , the head casting of Drosophila larva might represent an intermediate odour-tracking strategy purely based on spatio-temporal sampling. As we progressively delineate the logic of how sensory signals are encoded in the nervous system, we become in position to address the molecular, cellular and computational bases of active sampling and decision-making in goal-oriented behaviours. The recent advent of new technologies to conduct optogenetics in freely moving nematodes [41] should help us decipher how odour perception, motor behaviour and active sampling are intertwined in a feedback process. Fly stocks and transgenic strains Fly stocks were maintained on conventional cornmeal-agar molasses medium at 22 °C and kept in a 12 h dark–light cycle unless indicated otherwise. w1118 was used as a 'wild-type' control. We genetically engineered larvae with one class of functional ORNs—one ORN on each side of the head—by restoring the expression of Orco (previously termed Or83b ) in the Or42a -expressing ORNs [13] . Ectopic expression of Or42a was induced in all larval ORNs by driving the expression of UAS- Or42a with the Orco -Gal4 driver. The UAS- Or42a transgene was donated by Yelena Fishilevich and Leslie B. Vosshall. It was created by cloning full-length Or42a complementary DNA into a pUAST vector [42] and by generating transformants according to standard methods [16] . Unilateral Or42a -functional larvae were obtained by using an Orco UAS-flipout construct to stochastically restore the expression of Orco in the Or42a -expressing ORN [8] . These larvae where raised at 28.5 °C. Forty-eight hours after egg laying, larvae were subjected to a 15-min heat shock at 36 °C. Individuals were not pre-sorted by phenotypes before the behavioural experiments. After each behavioural experiment, the anterior tip of the larva was isolated, fixed in 4% formaldehyde solution and rinsed abundantly with PBS. The phenotype of each larva was then assessed by confocal microscopy based on the detection of GFP expression. Spectroscopy-based odour gradient reconstruction Odour-based experiments were conducted with ethyl butyrate (Sigma-Aldrich) at the highest level of purity. The odour was diluted in paraffin oil. Odour gradients were created in mini arenas composed of a stack of three 96-well plate lids. The odour source consisted in 10 μl odour loaded in one of the wells of the top lid. Odorant concentrations were measured in gas phase based on the fast-Fourier infrared spectroscopy method described in ref. 8 . Absorption of infrared light was quantified with a Tensor 27 (Bruker Optics) along the length and the width of the plate at a wave number of 1,758 cm −1 every 12 s (averages over 44 scans). The reconstructed gradient was computed from absorbance measurements averaged between one and five minutes on introduction of the odour in the plate. The topography of the two-dimensional gradient was inverted by a simple topographical method [8] . A shape-preserving piecewise cubic interpolation was applied to map the reconstructed odorant landscape on a two-dimensional 0.1 mm square-lattice mesh. Behavioural arena and animal preparation All behavioural experiments involved third instar foraging larvae tested during the day. Room temperature was kept between 22 and 24 °C and relative humidity fluctuated between 50 and 60%. A light pad (Slimlite Lightbox, Kaiser) illuminated the arena from above creating uniform daylight conditions. Larvae were washed by pouring a solution of 15% sucrose into each food vial. Individuals floating at the surface of the solution were transferred to the arena for behavioural tracking between 25 and 120 min after introduction of sucrose. Single animals were monitored for their chemoatic behaviour in a controlled odour gradient. Our chemotaxis assay consisted of a 3% agarose slab coating the top surface of a rectangular plate lid (Falcon, 353958). The bottom plate was covered by a conventional 96-well plate lid (Falcon, 353071) where an odour droplet was loaded in a single well. Immediately after the introduction of a larva in the arena, the top lid was inverted onto the agarose layer. Accordingly, larvae were exposed to an odour gradient in gas phase released from the odour source. The starting position of the animal and the location of the odour droplet coincided with the centre of arena in the near-source paradigm. The animal's initial orientation was random. In the approach experiment, the odour droplet was centred at the extremity of the plate. The larva started from the opposite side, facing the source. To prevent contamination, lids and agarose layers were not reused across experiments. Larvae were naïve and not reused across trials. Behavioural tracking lasted a maximum of five minutes and was interrupted as soon as the larva touched the plate walls. Tracking and image processing We developed custom-made tracking software written in Matlab (Mathworks). Recording of the larval body postures was carried from under the assay plates using a video camera (Stingray Camera, Allied Vision; Computer lens, 12–36 mm, 1:2:8, 2/3″ C) at a spatial resolution of 90 μm per pixel. Frames were acquired at 7 Hz and preprocessed online. Body shape images were cropped into a small bounding box enclosing the larva and, together with their absolute position in the arena system of reference, were saved for offline analysis. Following ref. 10 , the skeleton of the animal was extracted from the perimeter shape and its endpoints automatically classified as head or tail based on a proximity rule. The processing resulted in the conversion of raw images of the animal in the arena streamed directly from the camera into a temporal sequence of skeleton absolute positions, ordered from head to tail. Sensory-motor quantification Larval behaviour was monitored by projecting body postures on the plane of locomotion. From the temporal sequence of posture skeletons, we extracted the location of the animal's head, tail, midpoint and centroid. Raw trajectories were smoothed by a third-order polynomial fit using a 2-second time window. The animal's orientation and the direction of body motion were represented via the body angle, α, defined as the angle between body axis and the long axis of the plate. Such measure does not rely on an interpolation of the centroid trajectory and remains well defined even in the absence of spatial translation of the body. From the crossover observed in ensemble distribution of instantaneous reorientation rates ( Fig. 2b ), turning events we defined and trajectories automatically parsed into runs and turns. To avoid false positives, we considered turns whose duration was at least 1 s. The animal's lateral head bends were monitored via the head angle, θ , defined as the angle between the head and the body axes. This variable captures changes in posture, regardless of the body displacement. We used the turn-conditional distribution of the head angles to define head casts as lateral head movements of wide amplitude ( Fig. 2c ). Head casts are classified as belonging to a particular turn when they occur between 5 s before and 0.5 s after the turn initiation. Head casts and turns are treated as two distinct behaviours. Although the body necessarily follows the head during reorientation, a head cast does not imply the implementation of a turn. To measure the alignment of the body axis with the local odour gradient, we defined the bearing angle, β , as the relative angle orientation to the local direction of maximum concentration increase. We used the reconstructed odour gradient to map the position of the animal's head and centroid with the corresponding concentration in the arena. Markov model for action-perception state transitions A discrete-time first-order Markov model was developed based on four states: head cast towards low ( S LOW ), head cast towards high ( S HIGH ), turn towards low ( T LOW ) and turn towards high ( T HIGH ). Accordingly, the probability dynamics that the larva is found at time t in one particular state obeys a master equation. The corresponding probability transition matrix, M, was computed from the experimental sequence of state transitions. Individual matrix elements, m ij , were calculated by counting the total number of transitions observed from state j to state i . The transition probability matrix for wild-type larvae monitored in the near source paradigm was obtained by training the model. Based on a Monte Carlo algorithm, we used the transition probabilities of M to numerically simulate state transitions. For each state i , the interval [0,1] was partitioned into 4 segments and each segment was associated with one state: S LOW ↔[0, m 1i ], S HIGH ↔[ m 1 i , m 2 i ], T LOW ↔[ m 2i , m 3 i ], T HIGH ↔[ m 3 i , m 4 i ]. Each transition was assigned a random number picked between 0 and 1. The next state of the system was then defined by the interval to which the random number belonged. The number of simulated turns (1,243 events) was chosen equal to that of the experimental sequence of WT larvae. How to cite this article: Gomez-Marin, A. et al . Active sampling and decision making in Drosophila chemotaxis. Nat. Commun. 2:441 doi: 10.1038/ncomms1455 (2011).